From computational discovery to experimental characterization of a high hole mobility organic crystal For organic semiconductors to find ubiquitous electronics applications, the development of new materials with high mobility and air stability is critical. Despite the versatility of carbon, exploratory chemical synthesis in the vast chemical space can be hindered by synthetic and characterization difficulties. Here we show that in silico screening of novel derivatives of the dinaphtho[2,3-b:2′,3′-f]thieno[3,2-b]thiophene semiconductor with high hole mobility and air stability can lead to the discovery of a new high-performance semiconductor. On the basis of estimates from the Marcus theory of charge transfer rates, we identified a novel compound expected to demonstrate a theoretic twofold improvement in mobility over the parent molecule. Synthetic and electrical characterization of the compound is reported with single-crystal field-effect transistors, showing a remarkable saturation and linear mobility of 12.3 and 16 cm 2 V −1 s −1 , respectively. This is one of the very few organic semiconductors with mobility greater than 10 cm 2 V −1 s −1 reported to date. The field of organic electronics has gained tremendous interest in the last decade, motivated by flexible display [1] , photovoltaic [2] , [3] and sensor [4] , [5] , [6] , [7] applications. New materials are typically discovered experimentally, with theoretical characterization providing only post-facto justification of the observed device performance. In a few recent cases, however, theory in particular computational chemistry methods together with rational design techniques guided the synthesis of successful organic electronic materials for solar cell applications [8] and liquid crystals [9] . A priori screening of new materials and the prediction of the device performance would open vast opportunities for new materials design [10] . Theoretical prediction of high-performance novel organic semiconductor materials is hindered by the large number of factors influencing charge carrier mobility in thin-film devices; for example, synthetic methods, device geometry, contacts, device interfaces, thin-film growth, and molecular packing of the solid [11] . The challenge one faces is the choice of the 'right' molecule for synthesis. Although, π-extended compounds such as oligoacenes and oligothiophenes are known to be suitable as organic semiconductors, many factors on the molecular level, such as molecular reorganization energy, electronic structure and air stability must be optimized [12] . Moreover, the control of molecular properties is not sufficient for successful semiconductor design, as bulk properties (for example, orbital overlap, packing), and thus the delocalization of charges depend on the crystal structure. Therefore, accurate prediction of the molecular packing within the solid is crucial for computation of the magnitude [11] and anisotropy [13] of charge transport. Despite the recent advances in the crystal-structure prediction [14] , [15] , [16] , de novo prediction of organic crystal structures remains a challenging task [17] , [18] , [19] , [20] , but the related problem of optimizing the unit cell parameters is more tractable [17] , [21] . The difficulty arises from the fact that the sum of weak intermolecular forces such as van der Waals, H-bonding and π–π interactions determine the final packing structure. Although, there has been some recent success for the de novo prediction of crystal structures of small organic rigid molecules when the contents of the asymmetric unit is known [17] , [21] , the success of such predictions rely on highly accurate dispersion-corrected Density Functional Theory (DFT) methods that are precluded for the large extended π-conjugated heteroacenes. The theory of charge transport in organic semiconductors relies on two contributions. The first is the magnitude of the electronic coupling (transfer integral), which depends on the relative arrangement of the molecules in the crystal, whereas the second is the geometric relaxation of the molecule and its surroundings (reorganization energy) on movement of the charge carriers [11] , [22] . The former can be approximated as nearest-neighbour contributions, as the electronic couplings fall off rapidly with distance. The latter is mostly the energy change of a single molecule on charge addition/removal (intramolecular reorganization energy), because contributions from polarization of surrounding molecules is significantly smaller [23] , [24] . Previous calculations indicate that the high charge mobilities of pentacene and dinaphtho[2,3-b:2′,3′-f]thieno[3,2-b]thiophene ( 1 ) can be partially attributed to both strong electronic coupling interactions among neighbouring molecules and to a decrease of the hole intramolecular reorganization energy ( λ + ) [25] , suggesting that quantum-chemical calculations of these properties can be used to identify novel semiconductors. The present work was stimulated by the report of Yamamoto and Takimiya on a facile synthesis of 1 , with high hole mobility (2.9–3.1 cm 2 V −1 s −1 ) and stability in air [26] , [27] . Subsequent measurements on single-crystals of 1 yielded hole mobility of μ + =8.3 cm 2 V −1 s −1 (ref. 28 ) whereas Hall effect measurements by the same group provided an intrinsic hole mobility of 1.2 cm 2 V −1 s −1 (ref. 29 ). The stability of 1 in air, attributed to the deeper highest occupied molecular orbital (HOMO) level due to thienothiophene core [30] , is a significant improvement over pentacene, which readily undergoes many types of disproportionation reactions to generate impurities that decrease the mobility [31] . Compared with oligothiophenes, for example, the limited number of sulfur atoms in 1 results in smaller reorganization energies and thereby higher mobilities. Taken together, these factors have motivated previous work substituting different molecular fragments, such as thiophene and acene, to develop organic semiconductors with superior charge transport properties and air stability [12] , [30] . Molecule 1 is also a good model system for computational discovery of new materials. A computational search can use databases to limit possible candidates to commercially available or previously reported precursor candidates. Quantum chemical calculations are then performed to identify molecular derivatives exhibiting lower reorganization energies and higher transfer integrals than those of the parent compound. In this study, a computational screening procedure followed by synthesis and characterization led to single-crystal-based organic field-effect transistors (OFETs) of the new compound 2 that demonstrated a saturation region hole mobility of μ + =12.3 cm 2 V −1 s −1 and a linear region mobility of 16 cm 2 V −1 s −1 . This is one of the very few organic semiconductors that has exhibited mobility greater than 10 cm 2 V −1 s −1 . The study suggests that a computational screening approach can lead to the informed synthesis and characterization of novel organic materials for electronics applications. Screening procedure The screening procedure involved the following steps: design of potential derivatives of compound 1 from fused aromatics; computational screening for low reorganization energy candidates; crystal structure optimization; charge transport calculation to establish relative mobilities; selection of the most promising candidates with the highest mobility; synthesis; and finally, device fabrication and characterization. This approach was applied by theoretically screening seven new heteroacenes ( 2 – 8 , Fig. 1 ) to identify the most promising charge-transport materials, 2 and 7 . On the basis of the computational results, 2 was given priority over 7 because of higher transfer integral. It was subsequently synthesized, and single-crystal transistors were fabricated for charge transport characterization. 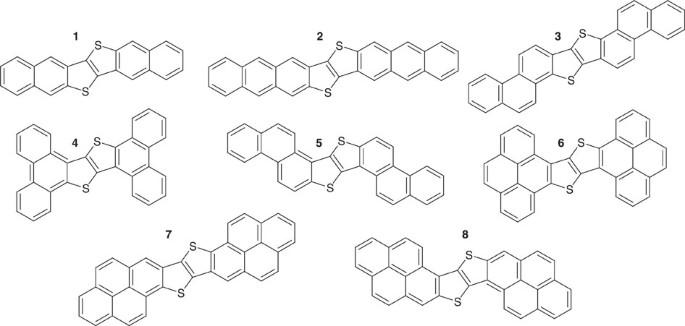Figure 1: The molecular structures of the targeted compounds. The structures of seven extra heteroacenes (2–8) derived from the parent dinaphtho[2,3-b:2′,3′-f]thieno[3,2-b]thiophene (1) computationally characterized as potential high-performance organic semiconductors. Figure 1: The molecular structures of the targeted compounds. The structures of seven extra heteroacenes ( 2 – 8 ) derived from the parent dinaphtho[2,3-b:2′,3′-f]thieno[3,2-b]thiophene ( 1 ) computationally characterized as potential high-performance organic semiconductors. Full size image Theoretical calculations We used a combined quantum-mechanical and molecular mechanics approach for the computational studies here, the details of which are presented in the Supplementary Methods . Here we first discuss results for 1 , to directly compare against known experimental values [27] . As shown in Table 1 , the calculated HOMO energy of 1 with the 6–311+G(d,p) basis is in reasonable agreement with the electrochemical cyclic voltametry measurement value of 5.44 eV (ref. 27 ). The calculated HOMO–LUMO (lowest unoccupied molecular orbital) gap, Δɛ , is also in reasonable agreement with the optically observed absorption edge of 3.0 eV, given that our calculation considers an isolated molecule in vacuum, whereas the experiment was performed on a crystal. The time-dependent density functional theory (TD-DFT) optical gap of 3.0 eV ( Supplementary Information ) is in excellent agreement with the experimental absorption spectrum. Use of the larger 6–311+G(d,p), basis set improves the orbital energies, but the reorganization energies are practically same for both basis sets. 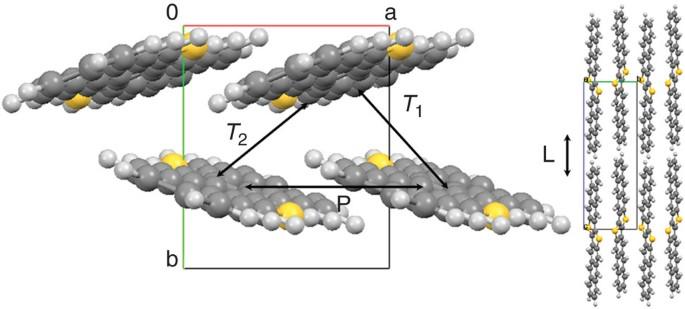Figure 2: Dimer type neighbours in the crystal structure of2. The projections on theab-(on the left) andbc-plane (on the right) of predicted crystal structure of2are shown. Unique transfer integrals are computed only for the transverse (T1andT2), parallel (P), and longitudinal (L) nearest neighbour pairs. To obtain a numerical estimate of the hole mobility for 1 , we used its experimental [27] as well as the predicted crystal structures ( Supplementary Table S1 ) to calculate the transfer integrals [19] , V + , the data are listed in Table 2 . In general, V + calculated for 1 is comparable to those of pentacene. However, the lower mobility for 1 results from the higher λ + ( λ + =0.128 eV for 1 , as compared with λ + =0.099 eV for pentacene [32] ) due to the exponential dependence of the hopping rate on this parameter, whereas quadratic power law dependence on the transfer integral, V + ( Supplementary Information , equation (1)). We also note that optimized crystal structures with charges calculated at the levels of Perdew–Burke–Ernzerhof [33] parametrization with the double numeric plus polarization basis [34] (PBE/DNP) -denoted 'DNP' and Becke three-parameter Lee–Yang–Parr functional [35] , [36] with the Gaussian basis (B3LYP/6–311+G(d,p)) [37] -denoted 'G' have slightly larger unit cells and lower predicted mobilities (1.64 cm 2 V −1 s −1 (DNP), 1.69 cm 2 V −1 s −1 (G)) compared with that of the experimental structure (1.90 cm 2 V −1 s −1 (xtal)). Table 1 Calculated energies of the target compounds. Full size table Table 2 Calculated structural and hole transport properties of selected molecules. Full size table Having established this approach with 1 , we next examined whether larger ring structures, such as 2 – 8 , could have better stability (that is, greater Δɛ , comparable or lower ɛ HOMO ) and lower λ + than 1 , and therefore yield higher performance OFET devices. Increasing the length of polyacenes leads to a decreasing Δ ɛ and λ + , so that a decrease in stability cancels any benefit from reduced λ + . However, as shown in Table 1, structures 3 , 4 , 5 , and 7 all have larger Δ ɛ than 1 . Given the inaccuracies of the gaps calculated by DFT in general and B3LYP in particular [38] , 6 , which is only 53 meV lower, may also be considered comparable to 1 . In addition, all of 3 – 7 have lower ɛ HOMO than 1 , adding support for their environmental stability. In contrast, both 2 and 8 have gaps that are lower than 1 by ~0.5 eV, with calculated HOMO–LUMO gaps between those of tetracene (Δ ɛ= 2.737 eV) and pentacene (Δ ɛ= 2.176 eV), and with ɛ HOMO comparable to tetracene ( ɛ HOMO =5.199) [39] . As 2 has a similar HOMO energy to tetracene, but with dramatically higher hole mobility ( vide infra ), it may be utilized to improve the hole-mobility limited [40] performance of tetracene/C 60 planar heterojunction photovoltaics. At the B3LYP/6–311+G(d,p) level of theory, 3 – 5 have λ + ~50 meV greater than 1 , comparable to that of naphthalene ( λ + =0.183 eV) [39] . Therefore, we conclude that these will have inferior carrier mobilities to 1 . In contrast, 6 has λ + comparable to 1 , while 2 and 7 have λ + that are 44 and 53 meV lower (respectively) than 1 , and moreover, lower than pentacene ( λ + =0.099 eV). Having identified 2 and 7 as the most promising candidates, in Table 2 columns, labelled '2(G)' and '7(G)', we show hole mobility results based on calculated crystal structures. As with pentacene and 1 , both show anisotropic mobility, with the strongest couplings for the T 1 dimer (see Fig. 2 ). In the case of 2 , the nearest-neighbour distances are comparable, and the transverse couplings slightly stronger than 1 , leading to a predicted μ + of 3.34 cm 2 V −1 s −1 , twice that of 1 . In the case of 7 , however, despite the much lower λ + , the transverse dimer couplings are weakened, leading to μ + slightly smaller than (but comparable to) 1 and pentacene (between 2.20 to 1.45 cm 2 V −1 s −1 ). This prediction of increased mobility and potential stability in air motivated the synthetic and device studies of 2 . Figure 2: Dimer type neighbours in the crystal structure of 2 . The projections on the ab- (on the left) and bc- plane (on the right) of predicted crystal structure of 2 are shown. Unique transfer integrals are computed only for the transverse ( T 1 and T 2 ), parallel (P), and longitudinal (L) nearest neighbour pairs. Full size image Synthesis and characterization The synthesis of 2 was carried out using a similar strategy as used for synthesis of 1 and its derivatives, Supplementary Figure S1 (refs 27 , 41 ). 2-Hydroxymethylanthracene ( S1 ) was first synthesized from anthraquinone-2-carboxylic acid [42] . S1 was then oxidized to the corresponding aldehyde, 2-anthraldehyde ( S2 ), using PCC in dichloromethane. The aldehyde S2 is photochemically unstable in solution; thus, the reaction involving this had to be carried out in dark. The thiomethyl group was selectively introduced to the 3-position of anthracene to yield 3-methylthio-2-anthraldehyde ( S3 ) using excess n -butyllithuim and dimethyldisulfide in presence of N , N , N ′, N ′-tetramethylethylenediamine. The olefin compound, trans-1,2-bis(3-methylthio-2-anthracen-yl)ethene ( S4 ), was synthesized using McMurry coupling. Owing to the poor solubility of these anthracene derivatives, purification of the S1 – S4 was achieved mainly via selective precipitation. The final ring closing reaction, to yield dianthracen-[2,3 -b :2′,3′ -f ]thieno[3,2 -b ]thiophene ( 2 ), was carried out in chloroform in presence of excess iodine. As the crude product was directly subjected to sublimation and a significant amount of product seemed to decompose in presence of reaction impurities at high temperature (~300 °C), the exact yield could not be determined. The subsequent sublimations and crystal growth experiments did not show material degradation. The UV-vis absorption spectrum of a thin film of 2 was collected ( Supplementary Fig. S2 ). The optical HOMO–LUMO gap is 2.2 eV as estimated from the onset of the absorption edge, which is 0.9 eV red-shifted from 1 (ref. 27 ). This is consistent with the calculated HOMO–LUMO gap, which predicts a 0.7 eV red-shift of 2 relative to 1 ( Table 1 ), and TD-DFT calculations which predict a 0.7 eV red-shift of the first excitation. The material was not soluble enough in organic solvents to allow for solution NMR or solution optical characterization. The HOMO of single crystals of 2 was estimated to be 5.2 eV from the ionization potential measured by photoelectron spectroscopy ( Supplementary Fig. S3 ) that is in excellent agreement with the calculated value of −5.2 eV at the level of B3LYP/6–311+G(d,p) theory. An X-ray diffraction pattern from crystals of compound 2 was collected at the Stanford Syncrotron Radiation Lightsource, at beamline 11-3 ( Supplementary Fig. S4 ). The unit cell structure was obtained by a least-square fitting method (homemade software employing a modified Levenberg–Marquardt algorithm) using the positions of 15 clearly measurable, overlap-free peaks in powder spectrum. The unit cell dimension is slightly smaller than the predicted one, similar as the case for compound 1 noted earlier. Using the experimental crystal structure, we re-calculated the transfer integrals and found much stronger coupling along the a- axis; V P increased from 0.0415 to 0.0687 eV whereas V T1 and V T2 are the same. Thus, the transfer integrals suggest that mobility along a- axis would be highest; we expect only a moderate anisotropy in the mobility in the ab -plane as all three transfer integrals are reasonably high. Ensuing calculated mobility of 3.36 cm 2 V −1 s −1 for the crystal is only slightly higher than the predicted value of 3.34 cm 2 V −1 s −1 . Thin-film devices Before studying the intrinsic transport characteristics of 2 through single-crystal devices, thin-film devices were fabricated for comparison. Because the yield of sublimation was low, performing more than two sublimation purification steps was not possible. Despite that, we are aware extra sublimation steps can significantly improve the performance of the device [43] . Nonetheless, thin-film transistors were fabricated by evaporation of a 40 nm layer of 2 on octadecylsilane-treated substrates at 95 °C, after which Au source and drain electrodes (40 nm) were deposited through a shadow mask. Atomic force microscopy demonstrated large two-dimensional growth of 2 , which is favourable for charge transport ( Supplementary Fig. S5 ). The transistors were measured in a glove box with N 2 atmosphere. The average mobility ( μ ) measured was 0.51±0.06 cm 2 V −1 s −1 with a threshold voltage ( V T ) of 37.9±1.3 V ( Supplementary Fig. S6 ). The on/off ratio was around 4×10 6 . The mobility of the evaporated thin films was lower than a comparable mobility for pentacene [44] or 1 (ref. 27 ) evaporated under the same conditions. We attributed the relatively low mobility value of 0.51 cm 2 V −1 s −1 to insufficient purification of the material. Additionally, the use of the crude, unpurified material resulted in an order of magnitude decrease in the mobility. There was no change in the thin-film transistor device performance following a six-month storage period in air, demonstrating the stability of 2 , even in the presence of thin-film impurities. Single-crystal devices To determine the charge carrier mobility in 2 , vapour-grown crystals were used to construct single-crystal field-effect transistors (SC-FETs). The use of vapour growth for the formation of single crystals was required due to the insolubility of 2 . An extra benefit of the use of crystal is the purification during crystal growth. We fabricated low-voltage SC-FETs utilizing the bottom-contact, bottom-gate geometry, with a novel cross-linked polymer dielectric recently reported by our group; namely PVP–HDA ( Supplementary Information ) [45] . The polymer allows for the use of low voltages and exhibits low dielectric leakage for device operation [46] . The polymer layer was formed according to our previously reported procedures, and Au bottom contacts were deposited through a shadow mask. The crystals were manually laminated onto the devices and individually screened for transistor behaviour. It should be noted that the formation of SC-FETs critically depends on the single-crystal morphology. In the case of 2 , the single crystals grew as ultra-thin plates; however, on average, the plates were limited in the lateral dimensions to ~100–400 μm. Additionally, owing to the thin nature of the plates, the larger crystals agglomerated together, making the selection of single-crystal candidates from the growth tube difficult. Nonetheless, the placement of the single crystals on the patterned electrodes usually resulted in the observation of transistor behaviour with high mobility. Indeed, from the twelve single crystals tested, seven exhibited mobilities of at or above 5 cm 2 V −1 s −1 . The mobilities measured in these devices that are made by hand-picking the crystals are, of course, expected to show a much larger variation in performance, because of crystal placement, contacts and crystal orientation. Additionally, the mobility of the crystal has been shown to be significantly improved with decreasing crystal thickness, thus, only thin, small plates were used [47] . Each crystal was subsequently examined under a cross-polarized microscope to ensure the crystal is not twinned or with multiple crystals ( Fig. 3 ). 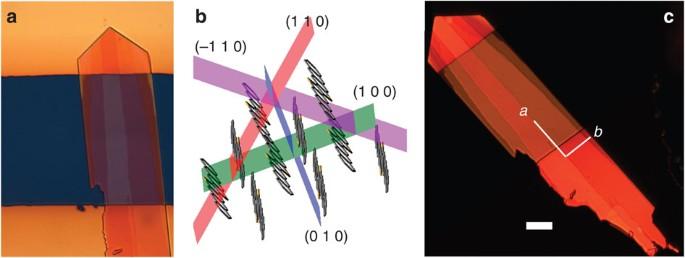Figure 3: Single-crystal optical and X-ray characterization. Shown here are the (a) optical micrograph and the (c) cross-polarized counterpart (under an angle of 45°) of the best performing device (μsat=12.3 cm2V−1s−1andμlinear=16 cm2V−1s−1) based on a single crystal of compound2. It is noted that we used an average of the length of each side of the crystal in contact with the electrodes as the channel width (W) for mobility calculation. The scale bar shown in pane (c) is 10 μm. (b) Crystal structure of2with labelled crystal planes used for facet identification, showing the molecular arrangement along thea-axis (0 1 0) plane, (blue). The angles of the facets as measured from the single crystal were matched to those calculated from the X-ray structure. The calculated and measured angles for the intersection of the (1 1 0) (red) and (0 1 0) (blue) planes were both 130.2°. The calculated and measured angles for the intersection of the (1 1 0) (red) and (−1 1 0) (purple) planes were 99.6° and 100.5°, respectively. Figure 3: Single-crystal optical and X-ray characterization. Shown here are the ( a ) optical micrograph and the ( c ) cross-polarized counterpart (under an angle of 45°) of the best performing device ( μ sat =12.3 cm 2 V −1 s −1 and μ linear =16 cm 2 V −1 s −1 ) based on a single crystal of compound 2 . It is noted that we used an average of the length of each side of the crystal in contact with the electrodes as the channel width ( W ) for mobility calculation. The scale bar shown in pane ( c ) is 10 μm. ( b ) Crystal structure of 2 with labelled crystal planes used for facet identification, showing the molecular arrangement along the a -axis (0 1 0) plane, (blue). The angles of the facets as measured from the single crystal were matched to those calculated from the X-ray structure. The calculated and measured angles for the intersection of the (1 1 0) (red) and (0 1 0) (blue) planes were both 130.2°. The calculated and measured angles for the intersection of the (1 1 0) (red) and (−1 1 0) (purple) planes were 99.6° and 100.5°, respectively. Full size image The best performance obtained for a laminated SC-FET was observed for the crystal shown in Figure 3 . The facets of the crystal are clearly visible and crystal is oriented such that the long-axis is along the electric field between source and drain electrode. Indexing of the crystal facets ( Fig. 3 ) confirms that the long axis of the crystal is the a -axis, consistent with the predicted high transfer integral direction. Thus, this crystal is aligned to exhibit the maximum device performance. Under cross-polarized light, no cracks or any other limiting factors for charge transport are visible ( Fig. 3c ). The near-perfect alignment with electric field and proper contact to the electrodes is likely the main reason why this particular device performs better compared with most other single-crystal devices. 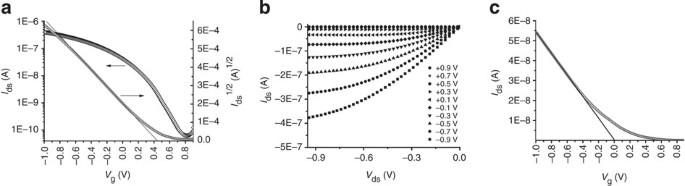Figure 4: Single-crystal device characterization. (a) Transfer characteristics in the saturation regime and (b) output curve of the single-crystal field-effect transistor of2with a field-effect mobility of 12.3 cm2V−1s−1. The drain-source bias (VDS) was −1.0 V, the threshold voltage (VT) was 0.44 V, and the on/off ratio was 6.4×103. (c) Transfer characteristics in the linear regime of the single-crystal field-effect transistor with a field-effect mobility of 16.0 cm2V−1s−1. TheVDSwas −0.1 V. The transfer and output characteristics of the device are shown in Figure 4 , below. The maximum mobility reached was 12.3 cm 2 V −1 s −1 in the saturation regime and 16.0 cm 2 V −1 s −1 in the linear regime using −0.1 V as the drain-source ( V DS ) bias ( Fig. 4c ). The on/off current ratio was 6.4×10 3 with a threshold voltage V T of 0.44 V. To ensure accuracy in the measurement, the capacitance of the dielectric was measured directly next to the placed single crystal as 68 nF cm −2 . The channel width/length ( W / L ) parameter (0.5) was extracted by measuring the single crystal under a digital microscope and taking the average of the two sides of the crystal in contact with the electrodes. The gate leakage for the device was on the order of 0.1 nA ( Supplementary Fig. S7 ). Both transfer and output characteristics show excellent scaling with the gate voltage, indicating there is no severe contact issues. It should be noted that the devices experienced less than 10% degradation in mobility after a period of six months storage in the ambient environment, attesting to the air stability of the compound. Moreover, during the submission of this manuscript, an independent study by the Takimiya group reported the synthesis and thin-film transistor characterization of 2 [48] . This paper demonstrated similar stability for thin-film devices with a lower observed mobility of 3.0 cm 2 V −1 s −1 . Previously, our group proposed a similar synthetic route within a published US patent [49] . Figure 4: Single-crystal device characterization. ( a ) Transfer characteristics in the saturation regime and ( b ) output curve of the single-crystal field-effect transistor of 2 with a field-effect mobility of 12.3 cm 2 V −1 s −1 . The drain-source bias ( V DS ) was −1.0 V, the threshold voltage ( V T ) was 0.44 V, and the on/off ratio was 6.4×10 3 . ( c ) Transfer characteristics in the linear regime of the single-crystal field-effect transistor with a field-effect mobility of 16.0 cm 2 V −1 s −1 . The V DS was −0.1 V. Full size image To establish an accurate comparison of the single-crystal result of 2 to that of the parent compound 1 , we fabricated several single-crystal devices utilizing the same device architecture described within the paper. This is necessary as variations in device fabrication could result in changes in device performance. To this end, within our studies, 1.19 cm 2 V −1 s −1 was the highest value of mobility for a single crystal of 1 ( Supplementary Fig. S8 ). This number agrees well with a recent report of the Hall mobility measured for 1 (ref. 29 ) Whereas this is approximately a factor of 10 lower than that obtained for 2 , the intrinsic value for the mobility of 2 needs to be evaluated by similar Hall effect studies. In summary, we have demonstrated a theoretical screening approach for the discovery of novel organic semiconductor cores before chemical synthesis. On DFT calculation of eight semiconductor cores, 2 was found to have lower hole reorganization energies than both 1 and pentacene. Charge transport modelling indicated that 2 would have a higher hole mobility than that predicted for 1 . On the basis of these calculation results, 2 was selected as a promising high mobility candidate. It was synthesized and characterized in single-crystal OFET devices. Single-crystal transistors demonstrated saturation region hole mobilities as high as 12.3 cm 2 V −1 s −1 and a linear region mobility of 16 cm 2 V −1 s −1 . This high mobility combined with high air stability (less than 10% degradation in SC-FET performance after a six-month period of storage in air), makes 2 a promising candidate for high-performance OFET applications. Future synthetic work will focus on the improvement of synthetic yield of 2 , and the introduction of pendant side chains and the synthesis and experimental characterization of 7 that is predicted to have similar performance to the molecule 1 . The development of more sophisticated theoretical models that go beyond the semiclassical regime, with the goal of bridging the gap between the predicted hopping-mechanism calculations and the measured mobility, is underway. This study suggests that computational screening is a viable approach for finding novel organic materials for electronics and photovoltaic applications. A high-throughput version of this screening of materials, by means of IBM's World Community Grid and the Clean Energy Project ( http://www.worldcommunitygrid.org and http://cleanenergy.harvard.edu ) is in progress (Olivares-Amaya R. et al ., unpublished work and Hachmann J. et al ., unpublished work). Strategies for predicting the carrier type based on single-molecular calculations can be used to screen for n-channel and ambipolar materials in addition to the p-channel materials studied here [50] . Computational methodology Geometries of the neutral ground state and radical cations were calculated at the B3LYP/6–31G(d,p) level of theory, followed by single-point calculations employing the valence-triple- ζ 6–311+G(d,p) basis set [35] , [36] , [51] , [52] for faster convergence as implemented in the Q-Chem software package [37] . The reorganization energies, shown in Table 1 , are calculated based on the usual four-point scheme [22] neglecting the outer sphere contributions to the total reorganization energy. Crystal structure prediction We performed crystal structure prediction only for the molecules 1 , 2 and 7 , because 2 and 7 are identified as promising candidates for OFET applications based on the isolated molecule properties. Because of the structural similarities of 2 and 7 to 1 , we hypothesized that the most probable packing motif would be a herringbone type with P2 1 similar to 1 . We modified the initial guesses of the unit cell parameters from 1 in accordance with the sizes of the molecules 2 and 7 , then performed rigid body optimization of the unit cell dimensions constructed from the calculated gas phase molecular structures. We employed the Dreiding [53] force field with ab initio point charges fit to the electrostatic potential, and optimized the unit cell using a combination of steepest descent, Newton–Raphson and quasi-Newton methods [19] . The long-range periodic electrostatic interactions were evaluated by Ewald sums. The results presented here are based on a lattice energy minimization of motionless molecules (that is, finite temperature effects are totally neglected). To validate this approach, we attempted to reproduce the experimental crystal structure of 1 . For 1 , the initial guess for the optimization was the experimentally determined unit cell. The effect of charges calculated by PBE/DNP [34] and B3LYP/6–311+G(d,p) levels of theory on the unit cell parameters of 1 are shown in Supplementary Table S1 , indicated by (DNP) and (G), respectively. Both yield comparable structure parameters to the experimentally determined unit cell, although B3LYP/6–311+G(d,p) charges have slightly better agreement with the experimental unit cell parameters and density. Consequently, the latter was used for the computations on 2 and 7 . All crystal prediction calculations were carried out with the Materials Studio Modules, Forcite and DMol [34] . Mobility calculations The mobility calculations were performed assuming diffusion of charges in the absence of an electric field, with charge carrier transfer rates obtained from the semiclassical Marcus theory [32] . Although this approach neglects tunnelling contributions to the mobility, which can significantly increase the hole mobility of highly purified polyacenes [43] , especially at low temperatures [54] , our present goal is to obtain a lower bound estimate of the performance for these materials in the presence of impurities, polymorphism, and temperature effects leading to carrier localization best described by a hopping model. Further description of the mobility calculations is provided in the Supplementary Information . Synthesis of compound 2 The complete synthetic route for compound 2 is included in the Supplementary Information . Dianthra[2,3-b:2′,3′-f]thieno[3,2-b]thiophene ( 2 ). A solution of S4 (0.18 g, 0.38 mmol) and iodine (4 g, 15.8 mmol) in chloroform (25 ml) was refluxed for 21 h. After cooling to room temperature, saturated aqueous sodium hydrogen sulfite solution (40 ml) was added, and the resulting precipitate was collected by filtration and was washed with water and chloroform. The crude product was purified by vacuum sublimation to provide a bright pink product. MS (MALDI) m/z= 440.17 (M+H + ), calcd m/z= 440.0693. Purification of materials Before use in thin-films or single-crystal growth both 1 and 2 were purified twice by sublimation using a three-temperature zone furnace (Lindberg/BlueThermo Electron) at a reduced pressure of 1×10 −4 Torr or less. Surface modification and thin-film device preparation is reported in the Supplementary information . Single-crystal device characterization The devices were tested in bottom contact geometry with crystals laminated across thermally evaporated gold contacts on the polymer dielectric. Previous studies on SC-FETs have established that to achieve maximum performance conformal elastomeric [55] or free-space dielectrics [56] should be employed. In this fashion, the dielectric acts as a passivated surface to the critical crystal interface as well as providing a conformal contact to the crystal. This lamination typically helps create an efficient contact with the bottom electrodes, and allows for efficient charge injection. The gold contacts were thermally evaporated in high vacuum at a rate of 1 Å s −1 while rotating the substrate holder. The electrode dimensions were defined by a shadow mask with a 50 μm channel length ( L ), and a W / L ratio of approximately 20. The W / L used in the mobility calculation for SC-FETs was determined from the individual crystals used. The SC-FET transistors were characterized using a Keithley 4200SCS and standard probe station setup in air. The thin-film transistors were characterized using the same probe setup in N 2 . Overall no significant difference between the performance in N 2 and in air was observed. Devices were tested in the saturation regimes and linear regimes with the device parameters extracted using the standard calculation techniques. The saturated field-effect mobility was calculated by plotting the square root of the source-drain current ( I DS ) versus gate voltage ( V GS ) and using the mobility equation from the saturated regime: The linear field-effect mobility was calculated by plotting the source-drain current ( I DS ) versus gate voltage ( V GS ) and calculating the slope m linear . The mobility was calculated according to the equation for the linear regime: The capacitance value of the polymer dielectric was evaluated using an Agilent E4980 precision LCR meter operating at 1 V and 1 kHz frequency. The capacitance was evaluated directly on the bottom contact electrodes that were used in the placement of the single crystal, to avoid discrepancies with polymer thickness. Electrodes of different dimensions on the polymer substrate were evaluated and the capacitance was confirmed to remain constant across the device. Crystal growth Single crystals of 2 were grown by the physical vapour transport method [57] at atmospheric pressure in semiconductor-grade argon at ~80 ccm; the details of this setup are described elsewhere [58] . The material formed two-dimensional platelets of varying quality. All platelets were pink/red, depending on crystal thickness. The single crystals of 1 were grown according to previously published literature procedures [28] . Surface characterization Atomic force microscopy was performed using a Digital Instruments Nanoscope IV operated in tapping mode (~320 kHz frequency, Si tip). Cross-linked poly(4-vinylphenol) (x-PVP) (refs 46 , 47 ). Poly(4-vinylphenol) (PVP, Aldrich, MW 25,000) was dissolved in propylene glycol monomethyl ether acetate (PGMEA) with ratio of 40 mg ml −1 . Separately, the cross-linker with 4,4′-(hexafluoroisopropylidene) diphthalic anhydride (HDA, Aldrich) was dissolved in PGMEA at a ratio of 4 mg ml −1 . Into a 2 ml solution of PVP, 2 μl of triethylamine was added, and the solution was shaken for a period of 30 s to ensure complete mixture. To this mixture, 2 ml of HDA solution was added, and the solution shaken to ensure complete mixture. Before spin coating, the blank silicon substrates were exposed to gentle UV-ozone treatment (Jelight Model 42) for 3 min to promote polymer adhesion. To form the thin dielectric film, a filtered (0.2 μm PTFE filter) dielectric solution (~200 μl) was deposited onto the desired substrate, and allowed to settle for a period of 30 s. The substrate was subsequently spun coated (using Headway Research spin coater) at 7,000 RPM for 1 min and then cured on a hot plate at 100 °C for 1 h. A second UV ozone treatment of the x-PVP layer (3 min) was followed by the spin-coated deposition of an extra x-PVP layer following the above procedure. The device was subsequently cured on a 100 °C hot plate for 4 h. How to cite this article: Sokolov, A.N. et al . From computational discovery to experimental characterization of a high hole mobility organic crystal. Nat. Commun. 2:437 doi: 10.1038/ncomms1451 (2011).